Nanosecond white-light Laue diffraction measurements of dislocation microstructure in shock-compressed single-crystal copper Under uniaxial high-stress shock compression it is believed that crystalline materials undergo complex, rapid, micro-structural changes to relieve the large applied shear stresses. Diagnosing the underlying mechanisms involved remains a significant challenge in the field of shock physics, and is critical for furthering our understanding of the fundamental lattice-level physics, and for the validation of multi-scale models of shock compression. Here we employ white-light X-ray Laue diffraction on a nanosecond timescale to make the first in situ observations of the stress relaxation mechanism in a laser-shocked crystal. The measurements were made on single-crystal copper, shocked along the [001] axis to peak stresses of order 50 GPa. The results demonstrate the presence of stress-dependent lattice rotations along specific crystallographic directions. The orientation of the rotations suggests that there is double slip on conjugate systems. In this model, the rotation magnitudes are consistent with defect densities of order 10 12 cm −2 . Although the shock compression of condensed matter has been a field of study for many decades [1] , [2] , [3] , [4] , [5] , [6] , our understanding of what occurs at the lattice level during the passage of a shock through a condensed matter system is woefully incomplete. It is well known that many simple metals, when shocked to high stresses under the constraint of uniaxial macroscopic strain, exhibit a peak stress–volume relationship (the ‘PV Hugoniot’) that closely follows the pressure–volume curve for hydrostatic compression. For this to occur, the material must have exhibited rapid plastic flow, which in many materials is expected to occur via the generation of defects (such as stacking faults or full dislocations), and their subsequent shear-stress-driven motion. From the theoretical standpoint, much has been learnt in recent years due to huge increases in computational capacity that have led to the capability to perform classical molecular dynamics simulations on systems with increasing sample size. Pioneering work in this area was performed by Holian et al . [5] , who demonstrated in simulations of single crystals of Lennard-Jonesium that large numbers of stacking faults were generated when shocks were applied along the [001] axis. Subsequent work employing potentials that better match the characteristics of real copper crystals [7] have also indicated that stacking faults are generated for shocks along [001], with full dislocations being seen in the case of shock compression along the other principal axes [8] , [9] . The generation of defects alone is not sufficient to relieve the shear stress, and it was observed in simulations by Bringa et al . [10] that a few tens of picoseconds may be required (for shocks of order a few tens of GPa) for the stress-driven motion of defects to relieve the shear stress. This work also demonstrated consistency with the classic equation of plasticity, developed by Orowan [11] —i.e., the plastic strain rate was found to be where ρ m is the density of mobile dislocations, b is the magnitude of the dislocations Burgers vector and v is their mean speed. Despite the insights that have been afforded by the large-scale computations mentioned above, direct in situ experimental evidence for what occurs during shock-induced plastic flow, even for the simple case of a single crystal shock compressed along a principal axis, remains elusive. Given that the fundamental understanding sought is of the physics that is occurring at the lattice level, the development of techniques of X-ray diffraction on nanosecond and sub-nanosecond timescales, with the X-ray pulse synchronized to the shock, appears a promising approach for such investigations. Indeed, such time-resolved X-ray diffraction (TXRD) methods have been used extensively to study shock phenomena for several decades [12] , [13] , [14] , [15] , [16] , [17] , [18] , [19] , [20] , with several notable successes, including the direct observation of the α−ε transition in shock-compressed iron [6] , [21] . Some progress in understanding rapid shock-induced plasticity has been made: diffraction of monochromatic X-rays from planes parallel and perpendicular to the shock propagation direction has directly detected elastic strain in both directions (which gives a measure of plastic strain, as the total strain (elastic plus plastic) perpendicular to the shock propagation direction in a uniaxially strained material is zero) [16] , [22] , [23] , [24] , [25] . Furthermore, broadening of the diffraction peaks observed in both shocked copper [25] , aluminium [26] and LiF [27] are consistent with large defect densities and/or lattice rotations. However, the monochromatic diffractions techniques employed, relying solely on the observation of broadening of a Bragg peak, could not provide any information on whether such lattice rotation took place along any specifically preferred directions. Here, we report on the use of a novel TXRD technique—nanosecond white-light Laue diffraction [28] —to record the first in situ measurements of lattice rotations, and their directions, in a shocked crystal. In contrast to TXRD methods previously employed, this method allows a large region of reciprocal space to be interrogated, and records a two-dimensional projection of the scattered intensity in that reciprocal space. We observe an increase in lattice rotation as a function of shock pressure, and deduce defect densities consistent with those seen in multi-million atom molecular dynamics simulations. Experimental set-up The experiments were performed at the Jupiter Laser Facility at Lawrence Livermore National Laboratory, using the JANUS high-power laser. The experimental layout is shown in Fig. 1 . Quasi-white-light X-rays, in the energy range of 3–10 keV, of 2 ns duration, are emitted from a laser-produced plasma, generated from a layered foil of mid-Z elements. This X-ray source was positioned 50 mm from the copper target, and collimated with pinholes such that an X-ray beam with divergence of order 4 × 10 −2 radians (and thus diameter of order 2 mm) was incident upon the target to be shocked. The back-reflected X-rays were recorded on Fujifilm image plates. The majority of the shocked targets were single crystals of Cu, of 10 μm thickness, of [001] orientation, over-coated with a 20-μm layer of parylene and a 300-nm flash coating of Al. Shocks were launched into the Cu single crystals by laser ablation of the parylene overcoat, using a pulse synchronized to the X-ray generating laser pulse. The pressure in the shocked crystals was determined by measuring the rear surface velocity of the thin crystals with the standard VISAR (velocity interferometer system for any reflector) technique [29] , [30] , [31] . The diameter of the laser spot used to shock the crystal was deliberately chosen to be smaller than the X-ray spot incident on the crystal—as will be seen in the diffraction images this allows the relative position of the two to be directly recorded. Further details of the set-up can be found in the Methods section. 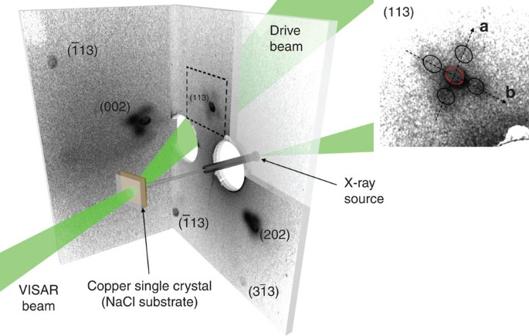Figure 1: Schematic diagram of the nanosecond white-light Laue set-up. The target is mounted at the centre of an image plate lined box, with the necessary apertures for the drive, X-ray and VISAR beams. The diffraction pattern shown in the figure is data from copper shocked along [001] at ~30 GPa, with the corresponding lattice planes labelled. Diffuse features are observed around the (002), (113) and (202) peaks, which are at lower energy where the X-ray source is brightest. The inset shows the (113) peak with the diffuse features marked. The axes a and b indicate rotation around the [100] and [010] crystal axes, respectively (two sides of the image plate box and the target and collimator supports have been removed for clarity). Figure 1: Schematic diagram of the nanosecond white-light Laue set-up. The target is mounted at the centre of an image plate lined box, with the necessary apertures for the drive, X-ray and VISAR beams. The diffraction pattern shown in the figure is data from copper shocked along [001] at ~30 GPa, with the corresponding lattice planes labelled. Diffuse features are observed around the (002), (113) and (202) peaks, which are at lower energy where the X-ray source is brightest. The inset shows the (113) peak with the diffuse features marked. The axes a and b indicate rotation around the [100] and [010] crystal axes, respectively (two sides of the image plate box and the target and collimator supports have been removed for clarity). Full size image X-ray Laue diffraction The nanosecond white-light Laue back-reflection patterns were recorded for shock pressures ranging from 17 to 50 GPa, with the X-ray pulse timed such that diffraction started between 0 and 0.5 ns before the start of the compression of the Cu crystal, and finished just before the shock had traversed the 10 μm thickness of the crystal (for 25 GPa the shock transits the 10 μm in ~2 ns). Figure 1 shows a section of the diffraction pattern for a shock at ~30 GPa. The brightness of the X-ray source is such that we record Laue spots for the basal plane, (002), as well as for the (202) and (113) planes (although certain of the (313) planes are visible, they are too weak to be used in the analysis to follow). From the data it can be seen that each main Laue spot is surrounded by four diffuse features, which we identify as being due to shock-induced micro-structural lattice rotation for the following reasons. The splitting of the Laue spot into four is seen on all the intense spots. The signal-to-noise ratio is typically greatest for the (002) peak ( Fig. 1 ) as this plane diffracts at lower energy (3.4 keV), where the X-ray source is brighter. As the shock propagates along [001], the position of the (002) peak does not change provided the plane normal remains parallel to the shock direction. Thus, only the magnitude of the reciprocal lattice vector changes, not the direction. This shows that the diffuse features are indeed due to a change in microstructure. Furthermore, as we see the diffuse features on three distinct Laue spots, widely separated in reciprocal space, we can determine whether they are consistent with diffuse scattering due to defects with a distinct periodicity, or due to rotations. If they were due to defects, then the data should be consistent with the addition of scattering vectors q to each of the three main recorded reciprocal lattice vectors of the compressed crystal, however, this is not the case. The four spots are, however, consistent with the assumption that at the micro-structural level the different regions of the single crystal have rotated positively or negatively around the [100] or [010] directions. The shock-generating laser spot was a square of 1 × 1 mm–smaller than the size of the X-ray spot on the crystal. Indeed, an image of the spot can clearly be seen in Fig. 2 –it is in the centre of the Laue spot, such that the bright surrounding area is diffraction from un-shocked crystal (we determined that the orientation of the diffuse features was independent of the orientation of the drive spot). The angle of rotation can be determined by measuring the position of the centre of the diffuse features with respect to the centre of the drive spot. These directions do not correspond to the broadening, which would be expected due to stacking faults, the 111 directions [32] . The angle of lattice rotation as a function of peak shock stress is shown in Fig. 3 , clearly demonstrating an increasing angle of rotation with increasing pressure. 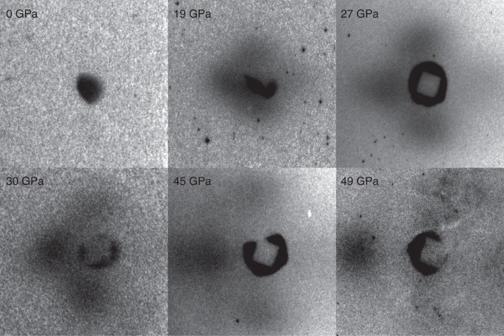Figure 2: (002) Diffraction peaks for six shots over a range of different pressures. As the shock pressure increases, the magnitude of the separation between the diffuse features and the driven region of the diffraction spot increases. Figure 2: (002) Diffraction peaks for six shots over a range of different pressures. As the shock pressure increases, the magnitude of the separation between the diffuse features and the driven region of the diffraction spot increases. 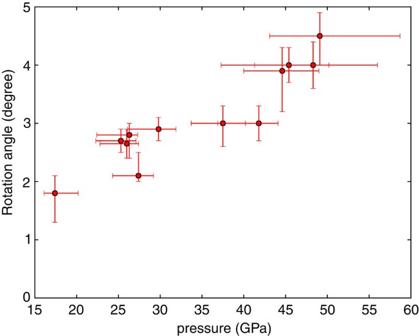Figure 3: Plot of lattice rotation angle against peak pressure. The rotation angle is measured for rotation of the lattice about the [100] and [010] directions. The mean is taken for all visible diffuse peaks, with error bars corresponding to the minimum and maximum fitted rotation angles. Pressure is determined using VISAR velocity profiles and the bulk copper Hugoniot. The velocity profiles were extracted from the VISAR interferograms using the Fourier transform method described by Cellierset al.31The mean velocity during the X-ray pulse is then converted to a pressure using the Hugoniot. The errors are calculated using the s.d. of the fringe shift, converting to velocity, and hence pressure, then taking the minimum and maximum values during the X-ray pulse. Full size image Figure 3: Plot of lattice rotation angle against peak pressure. The rotation angle is measured for rotation of the lattice about the [100] and [010] directions. The mean is taken for all visible diffuse peaks, with error bars corresponding to the minimum and maximum fitted rotation angles. Pressure is determined using VISAR velocity profiles and the bulk copper Hugoniot. The velocity profiles were extracted from the VISAR interferograms using the Fourier transform method described by Celliers et al . [31] The mean velocity during the X-ray pulse is then converted to a pressure using the Hugoniot. The errors are calculated using the s.d. of the fringe shift, converting to velocity, and hence pressure, then taking the minimum and maximum values during the X-ray pulse. Full size image The rotations we see under these conditions of uniaxial shock compression are consistent with the directions of rotation found under standard static tension/compression tests, where the directions perpendicular to the compression direction are constrained. In these static tests the lattice rotates with the slip plane normal approaching the compression axis [33] , [34] . For an fcc crystal, if the compression axis lies in the [001]−[101]−[111] triangle of a stereographic projection, the favoured slip plane is the (1 1) plane and the rotation of the lattice is equivalent to a rotation of the compression axis towards [1 1]. If the compression axis lies on the [001]−[101] symmetry line, slip is equally favoured on the (1 1) and (111) planes and the compression axis rotates towards [101] by so-called conjugate slip, as shown in Fig. 4 . For compression along [001], the four {111} planes are equally favoured. Slip on one of the planes causes a rotation towards the slip plane normal, and slip on the conjugate plane becomes more favourable. The rotations caused by conjugate slip are then equivalent to lattice rotations about the [100] and [010] axes [35] , as seen in our shock data. 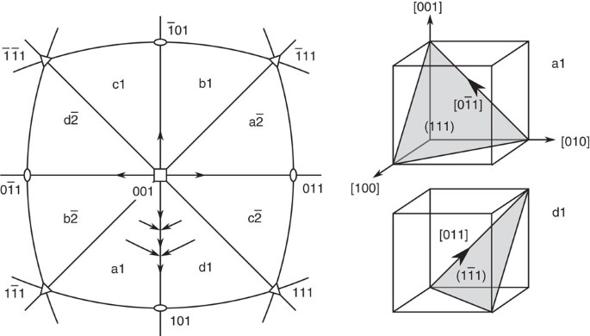Figure 4: Stereographic projection for cubic crystals. The slip systems for fcc crystals are indicated and the corresponding slip planes and directions given inTable 1. For a compression axis in the [001]–[101]–[111] triangle, the d1 slip system is favoured and resulting lattice rotation is equivalent to rotation of the compression axis towards the [11] direction, indicated by the arrows in the stereographic projection. On the [001]–[101] line, a1 and d1 are equally favourable and there is net rotation towards [101]36. The slip systems, a1 and d1, are illustrated in the right side of the figure. Figure 4: Stereographic projection for cubic crystals. The slip systems for fcc crystals are indicated and the corresponding slip planes and directions given in Table 1 . For a compression axis in the [001]–[101]–[111] triangle, the d1 slip system is favoured and resulting lattice rotation is equivalent to rotation of the compression axis towards the [1 1] direction, indicated by the arrows in the stereographic projection. On the [001]–[101] line, a1 and d1 are equally favourable and there is net rotation towards [101] [36] . The slip systems, a1 and d1, are illustrated in the right side of the figure. Full size image Within this model, the size of the measured rotation gives us some idea of the amount of slip occurring. For single slip, if we take a unit vector n normal to the slip plane and a unit vector m in the slip direction, the displacement tensor e ij , which describes the deformation, is given by e ij = am i n j , where a is the simple shear due to the slip [38] . This can be extended to two or more slip systems [38] , [39] . If we choose a conjugate slip system such as (111)[0 1] and (1 1)[011], we can calculate the simple shear for a given rotation angle. Under the assumption that the dislocations do not travel more than a few tens of nanometers (which is consistent with subsonic dislocation motion at the expected strain rates around 10 10 s −1 (ref. 4 ), we can infer dislocation densities of order 10 12 cm −2 . This order of magnitude is consistent with the defect densities predicted by Orowan's equation (1) and simulated in large-scale MD simulations, where defect densities of 10 12 −10 13 cm −2 are observed [10] , [40] , [41] . Table 1 The slip systems for an fcc crystal indicated in Figure 4 (ref. 37 ). Full size table In conclusion, our experimental results demonstrate shock-induced small-angle lattice rotations in a face-centered-cubic copper crystal shocked along the [001] axis. The distribution of the lattice rotations is about the [100] and [010] axes. The magnitude of the rotation increases with shock pressure, consistent with increased defect generation and slip. Lattice rotations of comparable magnitude have been observed in recovered shocked crystals [42] , and have also been shown to have an important role in dislocation dynamics simulations [43] , [44] . The rotation orientations suggest the action of conjugate slip systems and an inferred defect density of order 10 12 cm −2 . These measurements provide the first direct evidence on nanosecond timescales of stress-dependent lattice rotations in a shocked single crystal. X-ray diffraction In order to employ the Laue diffraction geometry in nanosecond timescales a broadband source is required rather than the quasi-monochromatic X-ray sources typically used in shock studies. The layered foil used to generate this source, as described earlier, consisted of Pd, Ag, Sn, Sm, CsI, Ti and V layers, which were irradiated at ~10 14 W cm −2 . Although broadband, the source has considerable spectral structure (as can be seen in [28] ), and thus although a projection of a wide volume of reciprocal space is recorded on the detector, the weightings of projections of particular regions in reciprocal space is not uniform as a function of distance from the origin. Drive Kinoform phase plates were used to smooth the drive laser spot to near uniform intensity, to produce a uniformly driven region of the target crystal. Typically the phase plate used, produced a 1 × 1-mm square spot on target, however the same results were observed using a circular drive spot. The energy in the driving laser pulse was varied between 20 and 100J. The target rear surface velocity was measured using a twin-bed line VISAR system, recorded on streak cameras typically covering a 20 ns sweep. The VISAR system was also used to synchronize the backlighter and drive beams to within 0.2 ns, after which the drive beam was kept at a fixed time and the backlighter beam delayed by a variable duration. The delay was adjusted over several shots such that the 2 ns pulse started 2 ns before the shock breakout at the rear surface of the Cu target. Variability of the drive energy resulting in earlier/later breakout meant that in some cases the backlighter pulse arrived up to 0.5 ns earlier or later. Targets The majority of targets used were 10 μm thick single-crystal copper, grown by vapour deposition on NaCl substrate. As described earlier, the drive laser side surface was coated with an ablation layer ~20 μm of parylene and a flash coating of aluminium. This allows the shock wave to steepen before entering the Cu crystal. Free standing crystals were obtained by dissolving the NaCl substrate in water, however, in general the NaCl substrate was not removed to act as a support. The same effect was observed for both cases. Transmission electron microscopy analysis of the undriven crystals showed an initial dislocation density of 10 9 cm −2 . Additionally data were collected for millimetre-thick copper single crystals grown via the Czochralski method, and coated with the same ablation layer. How to cite this article: Suggit M. J. et al . Nanosecond white-light Laue diffraction measurements of dislocation microstructure in shock-compressed single-crystal copper. Nat. Commun. 3:1224 doi: 10.1038/ncomms2225 (2012).